SiO and CH3OH mega-masers in NGC 1068 Maser is an acronym for microwave amplification by stimulated emission of radiation; in astronomy mega-masers are masers in galaxies that are ≥10 6 times more luminous than typical galactic maser sources. Observational studies of mega-masers can help us to understand their origins and characteristics. More importantly, mega-masers can be used as diagnostic tracers to probe the physical properties of their parent galaxies. Since the late 1970s, only three types of molecules have been found to form mega-masers: H 2 O, OH and H 2 CO. Here we report the detection of both SiO and CH 3 OH mega-masers near the centre of Seyfert 2 galaxy NGC 1068 at millimetre wavelengths, obtained using the IRAM 30-m telescope. We argue that the SiO mega-maser originated from the nuclear disk and the CH 3 OH mega-maser originated from shock fronts. High-resolution observations in the future will enable us to investigate AGN feedback and determine the masses of central supermassive black holes in such galaxies. Most of the SiO (silicon monoxide) masers in the Milky Way are known to occur around evolved stars and are collisionally pumped [1] , which reveal circumstellar envelope dynamics at high resolution [2] . A relatively low-level extragalactic SiO maser has been detected in the Large Magellanic Cloud with the same properties as SiO masers from the Milky Way sources [3] . Similarly, CH 3 OH (methanol) masers trace massive star-forming regions [1] , where Class I masers are pumped by collision and Class II masers are pumped by radiation [4] . Three species (H 2 O (ref. 5 ), OH (ref. 6 ) and H 2 CO (ref. 7 )) of extremely luminous masers, which are known as mega-masers [8] , have been found in galaxies. The 22.235 GHz H 2 O mega-maser provides a powerful probe of the accretion disk and supermassive black holes (SMBHs) in active galactic nuclei (AGNs), and enables the accurate determination of the angular-diameter distance of maser host galaxies, independent of standard candle arguments [8] , [9] . However, OH mega-masers are excellent tracers of heavily dust-embedded starbursts in the inner 100 pc of local ultra-luminous IR galaxies [8] , [10] . Numerous studies have been conducted to search for new mega-maser molecules for more than 30 years, without success [11] , [12] , [13] . A Class I extragalactic CH 3 OH maser has been recently found in NGC 253 that is 17 times more luminous than similar emissions near the galactic centre [14] and is still not a mega-maser. In this paper, we report the detection of millimetre SiO and CH 3 OH mega-masers at approximately the 5 σ level in the Seyfert 2 galaxy NGC 1068 using the IRAM 30-m telescope. Our results increase the number of known mega-maser molecules from three to five and may present new opportunities for studying AGN with the current powerful millimetre facilities, such as the Atacama Large Millimeter/submillimeter Array (ALMA). In Dec 2011, we used the IRAM 30-m telescope to observe NGC 1068, which hosts a circumnuclear gas disk (CND) within its inner 5′′ and two spiral arms that are rich in molecular [15] and dust emissions (see Fig. 1 ) [16] . We detected emissions of SiO J =2−1 ( υ =3) at 85.038 GHz and CH 3 OH 5 −1 -4 0 E at 84.521 GHz as mega-masers at the ~5 σ level. The SiO J =2−1 ( υ =3) emissions were detected at the velocity of 1,125 km s −1 with a FWHM (full width at half maximum) line width of only 1.5 km s −1 and the velocity of 1,362 km s −1 with a full width of ~8 km s −1 (see Fig. 2 ), whereas the CH 3 OH emission was detected at the velocity of 1,035 km s −1 with a FWHM width of ~84 km s −1 (see Fig. 3 ). 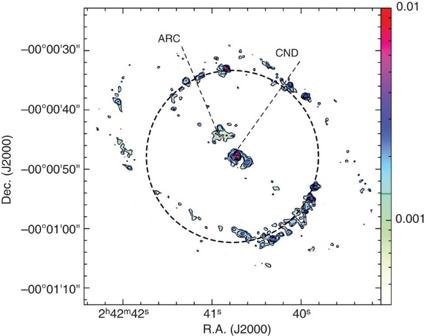Figure 1: Sub-millimetre dust emission in NGC 1068. Three hundred and forty-nine gigahertz dust continuum emission from ALMA observation16. The ‘CND’ is circumnuclear disk and ‘ARC’ is a ‘bow-shock’ arc defined by 349 GHz dust emission obtained by ALMA observation16. The dashed circle shows the beam of IRAM 30-m, while the colour scale is for the flux in the unit of Jy per beam shown with the colour bar in the right. Figure 1: Sub-millimetre dust emission in NGC 1068. Three hundred and forty-nine gigahertz dust continuum emission from ALMA observation [16] . The ‘CND’ is circumnuclear disk and ‘ARC’ is a ‘bow-shock’ arc defined by 349 GHz dust emission obtained by ALMA observation [16] . The dashed circle shows the beam of IRAM 30-m, while the colour scale is for the flux in the unit of Jy per beam shown with the colour bar in the right. 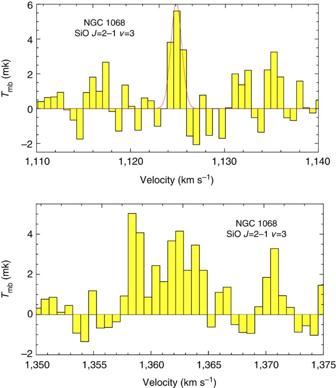Figure 2: SiO maser emissions detected in NGC 1068. Top: SiOJ=2−1 (υ=3) maser emission at the velocity of 1,125 km s−1in NGC 1068 detected with IRAM 30-m telescope, the noise level is about 0.93 mK at this velocity resolution (~0.69 km s−1), Thexaxis is the radio-defined velocity of SiOJ=2−1 (υ=3), while theyaxis is the main beam brightness temperature. The red line is the Gaussian fitting. Bottom: the same as that in the top but at the velocity of 1,362 km s−1. Full size image Figure 2: SiO maser emissions detected in NGC 1068. Top: SiO J =2−1 ( υ =3) maser emission at the velocity of 1,125 km s −1 in NGC 1068 detected with IRAM 30-m telescope, the noise level is about 0.93 mK at this velocity resolution (~0.69 km s −1 ), The x axis is the radio-defined velocity of SiO J =2−1 ( υ =3), while the y axis is the main beam brightness temperature. The red line is the Gaussian fitting. Bottom: the same as that in the top but at the velocity of 1,362 km s −1 . 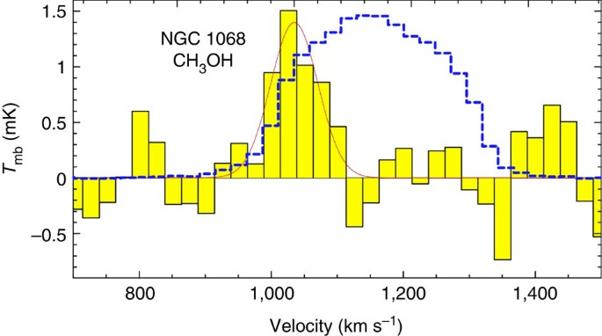Figure 3: CH3OH maser emission detected in NGC 1068. CH3OH 5−1-40Espectrum in NGC 1068 (black line and filled yellow histogram), smoothed to a velocity resolution of 24.9 km s−1, which gave the noise level of 0.37 mK. Thexaxis is the radio-defined velocity of CH3OH 5−1-40E, while theyaxis is the main beam brightness temperature. The blue dashed line represents the simultaneously obtained HCN 1-0 spectrum, which has been scaled down by a factor of 50, while the red line is the Gaussian fitting of the CH3OH 5−1-40Espectrum. Full size image Figure 3: CH 3 OH maser emission detected in NGC 1068. CH 3 OH 5 −1 -4 0 E spectrum in NGC 1068 (black line and filled yellow histogram), smoothed to a velocity resolution of 24.9 km s −1 , which gave the noise level of 0.37 mK. The x axis is the radio-defined velocity of CH 3 OH 5 −1 -4 0 E , while the y axis is the main beam brightness temperature. The blue dashed line represents the simultaneously obtained HCN 1-0 spectrum, which has been scaled down by a factor of 50, while the red line is the Gaussian fitting of the CH 3 OH 5 −1 -4 0 E spectrum. Full size image The only SiO J =2−1 ( υ =3) line that was detected in the Milky Way was a maser instead of a thermal emission [17] , and the detected SiO lines in NGC 1068 had much narrower line widths than the thermal lines (HCN 1-0, HCO + 1-0, etc. ); thus it was reasonable to assign the SiO line in NGC 1068 to a maser emission. However, the CH 3 OH 5 −1 -4 0 E line in the galactic sources could correspond to a maser emission, such as in DR21(OH) (ref. 18 ), or to thermal emissions, as in Orion [19] and W3(H 2 O) (ref. 20 ). Thermal emissions of four CH 3 OH lines (2 −1 -1 −1 E at 96.739 GHz, 2 1 -1 0 A + at 96.741 GHz, 2 0 -1 0 E at 96.744 GHz and 2 1 -1 1 E at 96.755 GHz) were detected as one line in an ALMA observation [21] because of the line broadening, which resulted in a flux of 1.05±0.03 Jy km s −1 in the nuclear region of NGC 1068. Each of the four CH 3 OH lines had a similar or an even higher Einstein A coefficient and a lower excitation condition than that of the 5 −1 -4 0 E transition [19] . The thermal flux of the 5 −1 -4 0 E line was <1/4 of that detected at 96.7 GHz in the nuclear region (that is, 0.26 Jy km s −1 ), which was to be expected; however, the detected CH 3 OH 5 −1 -4 0 E line flux was 0.53±0.1 Jy km s −1 and could not be explained as a pure thermal emission. Another piece of evidence, indicating that the 5 −1 -4 0 E line was not a pure thermal emission, was that the line was much narrower than the thermal lines (such as HCN 1-0), and line centre was shifted with respect to the thermal lines (see Fig. 3 ). Thus, we suggest that the detected CH 3 OH 5 −1 -4 0 E line in NGC 1068 originated from a maser emission instead of a thermal emission. The only source that has been reported for SiO J =2−1 ( υ =3) emissions is χ Cyg at a distance of 110 pc (ref. 22 ), with 0.23 and 0.37 K km s −1 at two epochs [17] , which yields an isotropic luminosity of ~0.2 Jy km s −1 kpc 2 . The isotropic luminosity of two velocity components of SiO J =2−1 ( υ =3) in NGC 1068 were 7.7±1.5 × 10 6 and 2.6±0.24 × 10 7 Jy km s −1 kpc 2 at velocities of 1,125 and 1,362 km s −1 , respectively, both of which match the criterion of a mega-maser as being ≥10 6 times more luminous than typical galactic maser sources [8] . Using the Orion molecular cloud(OMC)-2 as a typical galactic maser source of CH 3 OH 5 −1 -4 0 E (ref. 23 ), with a flux of ~200 Jy km s −1 , yields an isotropic luminosity of 34.3 Jy km s −1 kpc 2 , compared with 1.1±.02 × 10 8 Jy km s −1 kpc 2 for NGC 1068; thus this source can be considered to be a mega-maser of CH 3 OH 5 −1 -4 0 E . Our detected SiO maser exhibits extraordinary luminosity and has different properties from those of the Milky Way sources. The extremely narrow width of the detected SiO J =2−1 ( υ =3) line shows that it is impossible that the SiO emissions in NGC 1068 originated from more than hundreds of millions of the S-type Mira variable stars that have been detected in the Milky Way [17] . SiO masers in the Milky Way have been found with υ =1, 2 and 3 at multiple J transitions, whereas line intensities normally decrease with the increments in υ for the same J transition [17] . The SiO J =2−1 ( υ =1 and 2) transitions were also in the frequency range of our observation. We did not detect SiO J =2−1 ( υ =2) at similar noise levels to that of SiO J =2−1 ( υ =3), whereas we marginally detected SiO J =2−1 ( υ =1) at similar velocities (see Supplementary Fig. 3 ). This result shows that the excitation condition of the SiO molecules in NGC 1068 is different from that of the Milky Way sources and could be very close to that of the AGN, in which the gas temperatures are sufficiently high because the upper level energy of SiO J =2−1 ( υ =3) is equivalent to ~3,660 K above the ground state. Molecular gas with a high column density of an inverted population of SiO ( υ =3, J =2 and υ =3, J =1) is required to produce the detected mega-maser emission. The enhanced SiO abundance in the nuclear region [24] supplies SiO molecules for amplifying the emission under special excitation conditions. Extragalactic Class II CH 3 OH masers have been detected in Large Magellanic Cloud [11] , [25] , [26] , [27] , [28] and M 31 (ref. 29 ) with similar properties to those of star-forming regions in the Milky Way. Numerous studies have been conducted on searching for Class II CH 3 OH mega-masers over the past decades, without success [12] , [13] . Recently, a Class I extragalactic CH 3 OH maser was detected in NGC 253 at 36.2 GHz and exhibited an isotropic luminosity to more than one order of magnitude higher than that in the centre of the Milky Way [14] . Class II CH 3 OH masers are radiatively pumped and believed to be signposts of an early phase of massive star formation [29] , whereas Class I CH 3 OH masers originate from collisional excitation [4] . Both the CH 3 OH masers in NGC 253 at 36.2 GHz (ref. 14 ) and that we detected in NGC 1068 are hard to explain in terms of simple collections of thousands to millions of masers in massive star-forming regions and are Class I instead of Class II. It may be easier to increase the amplification length from collisional excitation than that from radiative pumping and thus easier to form mega-masers. Class I CH 3 OH masers at 84.5 and 36.2 GHz can be used together to determine the excitation conditions for the CH 3 OH molecule and further study the gas properties near AGN, such as NGC 1068, and nuclear starbursts, such as NGC 253. Both velocities of SiO emissions correspond to the velocities of the nuclear masers for the S1 component of the H 2 O mega-maser; the 1,125 km s −1 component is near the systemic velocity that is located toward the nuclear continuum peak of NGC 1068 for the H 2 O mega-maser in the nuclear disk, and the 1,362 km s −1 component is associated with the red component of the H 2 O nuclear maser that is located northwest of the continuum peak [30] . However, the velocity of CH 3 OH emission agrees well with the velocity of the C component of jet masers of the H 2 O mega-maser [30] . The different velocities and line widths of SiO and CH 3 OH lines show that these masers originated from different regions under different excitation conditions. It is likely that the SiO masers originated from the nuclear disk, whereas the CH 3 OH emissions originated from the shock front region where the nuclear jets (or outflows) interact with circumnuclear molecular clouds, which could be confirmed by future ALMA observation at the resolution of ~0.1′′. Thus, NGC 1068 is a unique case that exhibits luminous maser emissions of different molecules: H 2 O, SiO and CH 3 OH. Detailed studies of these mega-masers provide the opportunity to investigate the existence of SiO masers that require a pumping condition and the production of SiO molecules, which could result from AGN feedback in the nuclear region by X-ray radiation and/or shocks [16] , [24] . Maser spots near the nuclear regions can be observed using ALMA and located to a precision of several milliarcseconds, as has been achieved for H 2 O masers in NGC 1068 by VLA observations at A configurations with a beam size of ~0.08 arcsecond (ref. 30 ). Such observations can be used to study feedback from AGN in NGC 1068 to the innermost region of the molecular disk, whereas such studies are impossible for thermal SiO emission because of the absolute resolution and a limited brightness temperature. As CH 3 OH emissions are likely from the shock front region, a combination of SiO and CH 3 OH maser emissions can be used to study AGN feedback at sub-pc to ~100 pc scales. SiO mega-masers in nearby type II AGNs near the central SMBHs can be used as probes of AGN feedback and to directly measure the masses of the central SMBHs, as has been achieved using H 2 O mega-masers in nearby type II AGNs with <20 sources because of the limited sensitivity of current VLBI facilities [31] . Adopting the technique that has been used for H 2 O with VLA observation [30] , the structure of maser spots can be determined to ~2 milliarcseconds at the highest ALMA resolution of ~0.05′′. This structure corresponds to ~1 pc at a distance of 100 Mpc, which is primarily dominated by the gravity of the central SMBH. Observation and data reduction The observations were performed at the end of Dec 2011 using the IRAM 30-m telescope over 3 days under excellent weather conditions. The Eight MIxer Receiver (EMIR), the FTS backend and standard wobbler switching mode with ±120′′ offset at 0.5-Hz beam throwing, were used. The FTS at the wide band mode provided 8-GHz frequency coverage at 3-mm band and 195 kHz channel width spacing, which corresponds to ~0.69 km s −1 at 85 GHz. We determined whether the signal was from the sky frequency instead of from radio-frequency interference at the IF frequency or from the backend by separating the observations into two sub-configurations: on the first day, we set the H 13 CN 1-0 (86.340176 GHz) at the centre of the lower outer part of the EMIR, while we set the H 13 CO + 1-0 (86.754288 GHz) at the centre of lower outer part of the EMIR for the other two days. The total observation time was ~27 h, including tuning, pointing, focusing and the overhead of wobbler switching, which resulted in an effective on+off source time of ~15 h. The data were reduced with the CLASS package of GILDAS. We checked the data quality of each spectrum, which was read out every 12 min. All of the spectra exhibited good baseline and were thus all used in scientific analysis. The three SiO j =2−1 ( υ =1, 2, 3) maser lines and the SiO J =2−1 ( υ =0) thermal line were within the frequency range of our observation (~84–92 GHz). The typical system temperature during the observations was ~110 K. We averaged all of the spectra with the weight of the on-source time for final analysis, and we obtained averaged spectra for the two frequency tunings. Supplementary Figure 1 shows the final averaged spectrum using all of the data with an 8-GHz wide frequency coverage, which was only subtracted by a first-order baseline fitting and smoothed to a velocity resolution of ~24.3 km s −1 . Identification of SiO emission features The SiO J =2−1 ( υ =0, 1, 2, 3) lines were within the frequency range of our observation. Our data for the thermal line ( υ =0) were consistent with previous results that were detected using the IRAM 30-m telescope [32] , [33] and the IRAM PdBI [24] ; no reports of observations of masers lines could be found in the literature. Among the three transitions, we found that the strongest emission feature of the peak brightness temperature corresponded to SiO J =2−1 ( υ =3) at a velocity of 1,125 km s −1 , with the velocity-integrated flux of ~5 σ , which was obtained using a single Gaussian profile fitting. We confirmed that the signal corresponded to the frequency of SiO J =2−1 ( υ =3) and was not a radio-frequency interference at the IF frequency or a feature from a bad bandpass of the backend, by comparing the spectra from two different frequency tunings (see Supplementary Fig. 2 ): a SiO J =2−1 ( υ =3) emission was detected at the velocity of 1,125 km s −1 for both tunings. There was also an emission feature at the velocity of 1,125 km s −1 for the SiO J =2−1 ( υ =1) line (see Supplementary Fig. 3 ) at ~3.5 σ level, whereas no signal was detected at a similar velocity for SiO J =2−1 ( υ =2). On the basis of the detection results at different frequency tunings and the emission of the υ =1 line, we posit that the emission of SiO J =2−1 ( υ =3) at the velocity of 1,125 km s −1 was a real emission from NGC 1068. Another emission feature of the SiO J =2−1 ( υ =3) line was detected at the velocity of 1,362 km s −1 , with a slightly weaker peak brightness temperature but a larger velocity-integrated flux than that at the velocity of 1,125 km s −1 ; the counterpart of SiO J =2−1 ( υ =1) was also detected at the similar velocity (see Supplementary Fig. 3 ). This source was located at a galactic latitude of −51.9° at which it would be almost impossible to receive strong molecular emissions from the Milky Way. The line survey toward Sgr B2 and Orion-KL [34] shows that the only possible assignment for the SiO J =2−1 ( υ =3) at velocities of 1,125 and 1,362 km s −1 were c -C 3 H 2 at the frequency of 84.727691 GHz with velocities of 26.7 and 264.1 km s −1 . However, the absence of c -C 3 H 2 emission at the frequency of 85.338906 GHz with similar velocity, which is approximately three times stronger than the emission at the frequency of 84.727691 GHz in Sgr B2 and Orion-KL [34] , means that such emissions could not have originated from a Milky Way source. Estimation of isotropic luminosities of SiO and CH 3 OH mega-masers The isotropic luminosities were calculated by multiplying the flux densities (in units of Jy km s −1 ) by the squares of the distances from the sources. We calculated the isotropic luminosity of the SiO J =2−1 ( υ =3) emissions in χ Cyg, to be 0.3 K km s −1 × 54 Jy K −1 × 0.11 2 kpc 2 =0.196 Jy km s −1 kpc 2 , using a conversion factor of 1 K ≃ 54 Jy at 86 GHz (ref. 17 ). Our detections of SiO J =2−1 ( υ =3) were 8.86±1.76 mK km s −1 at 1,125 km s −1 using a single component Gaussian fit, and 29.4±2.7 mK km s −1 at 1,362 km s −1 , by integrating the velocity using the task ‘print area’ in CLASS from 1,357 to 1,365 km s −1 . Using a conversion factor of 4.2 Jy K −1 for the IRAM 30-m at 86 GHz and a distance of 14.4 Mpc (ref. 30 ), we obtained (8.86±1.76) × 4.2 × 14.4 2 × 10 3 =(7.7±1.5) × 10 6 Jy km s −1 kpc 2 for the 1,125 km s −1 component and (29.4±2.7) × 4.2 × 14.4 2 × 10 3 =(2.6±0.24) × 10 7 Jy km s −1 kpc 2 for the 1,362 km s −1 component. Using the same conversion factor, we obtained an isotropic luminosity of CH 3 OH of (1.1±0.2) × 10 8 Jy km s −1 kpc 2 at 125.1±24.7 mK km s −1 using a single component Gaussian fitting and we used a distance from Orion of 414 pc (ref. 35 ) to obtain an isotropic luminosity of CH 3 OH in the OMC-2 of 34.3 Jy km s −1 kpc 2 . Number of SiO mega-masers in local type II AGN available using ALMA Local Seyferts and LINERs were analysed using the CfA Redshift Survey catalogue, as a magnitude-limited sample with 82 sources [36] . Using the catalogue of galaxies that is classified on the CfA Redshift Survey website ( https://www.cfa.harvard.edu/dfabricant/huchra/zcat/ ), we found 110 Seyfert II galaxies with velocities below 7,300 km s −1 , which correspond to ~100 Mpc and can be revealed to 1 pc (2 milliarcseconds) using the ALMA. The sources in the CfA Redshift Survey were with δ >−2.5° and the ALMA can be used to observe sources with at least δ <+25°; thus, we can expect that over 150 Seyfert II galaxies within 100 Mpc could be observed using the ALMA. Including other type II AGNs, over 20 sources could be available to estimate the masses of SMBHs using the ALMA observations of SiO masers for the fraction of ~10%. How to cite this article : Wang, J. et al. SiO and CH 3 OH mega-masers in NGC 1068. Nat. Commun. 5:5449 doi: 10.1038/ncomms6449 (2014).